Solution-based circuits enable rapid and multiplexed pathogen detection Electronic readout of markers of disease provides compelling simplicity, sensitivity and specificity in the detection of small panels of biomarkers in clinical samples; however, the most important emerging tests for disease, such as infectious disease speciation and antibiotic-resistance profiling, will need to interrogate samples for many dozens of biomarkers. Electronic readout of large panels of markers has been hampered by the difficulty of addressing large arrays of electrode-based sensors on inexpensive platforms. Here we report a new concept—solution-based circuits formed on chip—that makes highly multiplexed electrochemical sensing feasible on passive chips. The solution-based circuits switch the information-carrying signal readout channels and eliminate all measurable crosstalk from adjacent, biomolecule-specific microsensors. We build chips that feature this advance and prove that they analyse unpurified samples successfully, and accurately classify pathogens at clinically relevant concentrations. We also show that signature molecules can be accurately read 2 minutes after sample introduction. Electronic readout of the presence of specific biological molecules in solution represents a powerful means to detect disease-related markers [1] , [2] , [3] , [4] . In particular, highly sensitive and specific methods have been developed to detect nucleic acids [5] , [6] , [7] , [8] , [9] , [10] , [11] , [12] , [13] , proteins [14] , [15] , [16] , [17] , [18] and small molecules [19] , [20] , [21] , [22] , using electrochemical readout, and it has been shown that the robustness of electrochemistry allows accurate detection to be done in the presence of heterogeneous, unpurified samples [20] , [23] , [24] , [25] . Numerous studies documenting the application of electrochemical sensing to cancer [17] , [23] , [26] , [27] and infectious disease [25] , [28] markers have illustrated the promise of this strategy for future clinical diagnostics, and the cost-effectiveness of the simple instrumentation needed for analysis further enhances the appeal of electrochemical detection for further development [1] . Arrays of serially addressed biosensors can be fabricated to work in conjunction with electrochemical reporter systems, enabling multiplexing and detection of several analytes simultaneously [29] . However, the need for independently addressed electrical contacts corresponding to each sensor, as well as reference and counter electrodes, requires that highly multiplexed arrays employ an active multiplexing strategy. The additional complexity of integrated active electronics explains why, before this work, electrochemical biodetection reports describe studies that employ very low levels of multiplexing [5] , [6] , [7] , [8] , [9] , [10] , [11] , [12] , [13] , [14] , [15] , [16] , [17] , [18] , [19] , [20] , [21] , [22] , [23] , [24] , [25] , [26] , [27] , [28] , [29] . Here we create distinct columns of connected biosensors, perpendicular to which we array distinct rows of electrochemical solution. Using this two-dimensional array of electrodes, we programme transient, solution-based circuits that permit individual analysis of sensors using shared contacts. This approach allows a much higher level of multiplexing than was attainable previously using a small set of contacts. We apply this advance towards the detection of panels of pathogenic bacteria and antibiotic-resistance markers. Overview of approach The solution circuit chip (SCC) is depicted in Fig. 1 . It consisted of 100 working electrodes (WEs) with 30 off-chip contacts. It included 20 common WEs and 5 counter/reference (CE/RE) electrode pairs, with 25 probe wells to facilitate manual probe deposition and 5 separate liquid channels ( Fig. 1a ). We defined templates for the sensing regions of the WEs by opening 5 μm apertures ( Fig. 1c ) in the top passivation layer. By restricting growth within these apertures, we then grew micron-sized tree-like electrodes via electrodeposition, resulting in nanostructured microelectrodes that protrude from the surface and reach into solution. It was previously shown that the micron-sized scale of the protruding electrodes increases the cross-section for interaction with analyte molecules [30] , whereas the nanostructuring maximizes sensitivity by enhancing hybridization efficiency between tethered probe and the analyte in solution [31] . Here these structures are being used to enable the creation of layered, insulated electrode arrays ( Fig. 1d ). 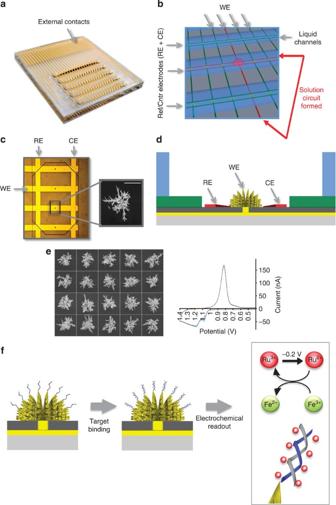Figure 1: The solution circuit chip. (a) An SCC featuring 5 liquid channels containing 20 sensors each. (b) An SCC featuring common WEs, and counter and reference electrode pairs (CE and RE) that can be activated in sets to form solution-based circuits (red). (c) Optical image of single probe well with 4 WEs. Inset: a scanning electron microscopy(SEM) image of a nanostructured microelectrode. Scale bar, 50 μm. (d) Cross-section looking down liquid channel of a sensor on a SCC: glass substrate (light grey), common WE (yellow), SU-8 passivation/aperture layer (dark grey), CE/RE (red), SU-8 probe wells (green) and SU-8 liquid channel barrier (blue). (e) Sensor-to-sensor comparison of SEM images and acid stripping scans for 20 sensors. Although morphological differences may exist, the surface areas of the sensors are highly consistent, as evidenced by the low levels of s.e. (blue error bars) observed for scans of the 20 sensors conducted in acidic solution. Gold oxide is formed at 1.05 V–1.3 V and reduced at 0.85 V. (f) Electrochemical nucleic acid assay scheme. PNA probes are immobilized on microsensors, and in the presence of a complementary target the electrostatic charge on the sensors is increased. This charge change is read out in the presence of Ru(NH3)63+and Fe(CN)63−, a mixture that yields currents that report on the amount of nucleic acid bound to the sensor. Figure 1: The solution circuit chip. ( a ) An SCC featuring 5 liquid channels containing 20 sensors each. ( b ) An SCC featuring common WEs, and counter and reference electrode pairs (CE and RE) that can be activated in sets to form solution-based circuits (red). ( c ) Optical image of single probe well with 4 WEs. Inset: a scanning electron microscopy(SEM) image of a nanostructured microelectrode. Scale bar, 50 μm. ( d ) Cross-section looking down liquid channel of a sensor on a SCC: glass substrate (light grey), common WE (yellow), SU-8 passivation/aperture layer (dark grey), CE/RE (red), SU-8 probe wells (green) and SU-8 liquid channel barrier (blue). ( e ) Sensor-to-sensor comparison of SEM images and acid stripping scans for 20 sensors. Although morphological differences may exist, the surface areas of the sensors are highly consistent, as evidenced by the low levels of s.e. (blue error bars) observed for scans of the 20 sensors conducted in acidic solution. Gold oxide is formed at 1.05 V–1.3 V and reduced at 0.85 V. ( f ) Electrochemical nucleic acid assay scheme. PNA probes are immobilized on microsensors, and in the presence of a complementary target the electrostatic charge on the sensors is increased. This charge change is read out in the presence of Ru(NH 3 ) 6 3+ and Fe(CN) 6 3− , a mixture that yields currents that report on the amount of nucleic acid bound to the sensor. Full size image By patterning channels on the SCC, we created separate liquid compartments ( Fig. 1a ). WEs are multiplexed on common leads such that they are physically isolated because of the air/water interface in liquid channels separating them. Reference and counter electrodes are routed along the liquid channels. The electrical isolation of the reference and counter layers from the WEs within the SCC, and the ability to bring the electrodes into contact at specific positions using the liquid channels, are the essential elements that allow solution-based circuits to be formed. The contacts made through the conductive solution allow transient circuits to be formed and allow individual contacts to address many sensors in series. The patterned microsensors are functionalized with peptide nucleic acid (PNA) probes specific to regions of targeted pathogens ( Fig. 1f ). Electrodes are exposed to samples of interest and binding occurs if a target nucleic acid is present. To detect positive target binding we use an electrocatalytic reporter pair [32] comprising Ru(NH 3 ) 6 3+ and Fe(CN) 6 3− . Ru(NH 3 ) 6 3+ is electrostatically attracted to the phosphate backbone of nucleic acids bound near the surface of electrodes by probe molecules and is reduced to Ru(NH 3 ) 6 2+ when the electrode is biased at the reduction potential. The Fe(CN) 6 3− present in solution auto-oxidizes Ru(NH 3 ) 6 2+ back to Ru(NH 3 ) 6 3+ , which allows for multiple turnovers of Ru(NH 3 ) 6 3+ and generates an electrocatalytic current. The difference between pre-hybridization and post-hybridization currents are used as a metric to determine positive target binding. Characterization of the SCC The SCC was fabricated using a series of simple lithographic steps followed by the electrodeposition of three-dimensional microsensors. The electrodeposition process produces sensors with somewhat variable nanoscopic morphologies, but as it is programmed to deposit the same number of gold atoms in each structure, it produces sensors with surface areas that vary by less than 10% ( Fig. 1e ). We employed electrochemical analysis to determine whether SCCs provided the necessary level of electrochemical isolation. We also devised a spectroscopic approach to confirm the isolation analysis. Cyclic voltammetry of ferrocyanide was used to evaluate electrochemical characteristics of SCCs versus standard serially connected chips ( Fig. 2a ). We observed that SCCs have nearly identical electrochemical signals to serially wired chips. It is noteworthy that grounding of all other unbiased counter, reference and working electrodes is required to eliminate crosstalk, as evidenced by the differential pulse voltammetry scans of ferrocyanide with and without the grounding of these electrodes ( Fig. 2b ). To further investigate whether signals from adjacent liquid channels were picked up by individual sensors, we added ferrocyanide adjacent to channels and monitored the effect on the signals obtained ( Fig. 2c ). It was observed that when ferrocyanide is added to an adjacent channel, there is minimal perturbation of the signal of ferrocyanide within the channel of interest. The effects of repeated scanning were also explored and were found to be minimal (data not shown). 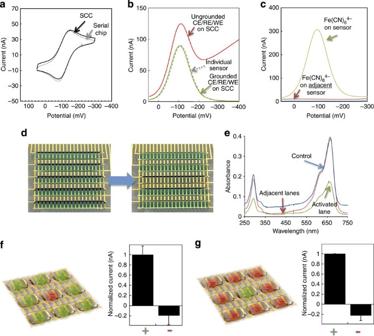Figure 2: Electrochemical validation of the SCC. (a) Cyclic voltammograms collected with standard chips with individually addressable electrodes and SCC electrodes in 2 mM ferrocyanide. (b) Differential pulse voltammetry of biased WE and CE+RE solution circuit in 2 mM ferrocyanide when unbiased CE, RE and WEs are ungrounded (red) and grounded (green) versus standard serially connected WE (dotted gray). (c) Differential pulse voltammetry of 2 mM ferrocyanide within liquid channel (green) and on adjacent liquid channels (red) of interest. (d) Evaluation of cross-talk by monitoring MB electrochemical bleaching. Middle channel was activated. (e) MB absorbance measurements for middle and adjacent lanes of SCC. (f) Analysis of signals obtained when sensors that are positive or (g) negative for a target sequence are surrounded by sensors yielding the opposite result. Figure 2: Electrochemical validation of the SCC. ( a ) Cyclic voltammograms collected with standard chips with individually addressable electrodes and SCC electrodes in 2 mM ferrocyanide. ( b ) Differential pulse voltammetry of biased WE and CE+RE solution circuit in 2 mM ferrocyanide when unbiased CE, RE and WEs are ungrounded (red) and grounded (green) versus standard serially connected WE (dotted gray). ( c ) Differential pulse voltammetry of 2 mM ferrocyanide within liquid channel (green) and on adjacent liquid channels (red) of interest. ( d ) Evaluation of cross-talk by monitoring MB electrochemical bleaching. Middle channel was activated. ( e ) MB absorbance measurements for middle and adjacent lanes of SCC. ( f ) Analysis of signals obtained when sensors that are positive or ( g ) negative for a target sequence are surrounded by sensors yielding the opposite result. Full size image A non-electrochemical strategy was also pursued to verify independently that the solution circuits were formed as desired, and to study any evolving leakage over longer time periods. To investigate electrochemical isolation using a spectroscopic approach we utilized methylene blue (MB), which can be electrochemically reduced to a colourless form ( Fig. 2d ). MB was loaded into all liquid channels, and WEs within the middle channel of the chip were held at the reduction potential of MB for 1 h. Visual evidence of the reduction of MB was observed exclusively in the selected channel, providing a qualitative measure of electrical isolation. Measurements of the absorbance ( Fig. 2e ) of each channel quantitatively confirmed that the significant loss in MB absorbance is detected in the middle lane only. To investigate whether signals from adjacent channels would interfere with our electrochemical nucleic acid assay, we investigated different orientations of sensors that would yield positive and negative electrochemical responses in the presence of a target DNA sequence. A small area of sensors was functionalized with a PNA probe sequence that would not bind a specific target DNA sequence, and this area was surrounded by sensors functionalized with a PNA probe that would bind the DNA target ( Fig. 2f ). On this chip, a large positive signal change was obtained with the positive sensors, and a small negative signal change was observed on the much smaller number of negative sensors. This indicates that with the nanoampere levels of current generated during sequence analysis, crosstalk between sensors does not influence the results obtained. When trials were conducted that reversed the positions of the positive and negative sensors, the expected reversed results were obtained ( Fig. 2g ). These results indicate that the solution-based circuits are indeed suitable for multiplexed sequence detection. Detection of urinary tract infection pathogens A compelling application for electrochemical analysis is the identification and classification of pathogens. Infectious disease can be difficult to diagnose accurately, because symptoms caused by different pathogens can be quite similar. However, it is important that a causative organism is identified correctly before a treatment is selected. We therefore elected to adapt the multiplexing capabilities of our chips to look for many different types of pathogens, and to also probe for antibiotic resistance. A set of PNA probes were designed, synthesized and tested, and validated for sensitivity and specificity ( Fig. 3 ). It is these probes that make individual sensors specific for pathogens, as they are targeted to unique sequences within the genomes of the organisms. The probe set developed covered 90% of the common urinary tract pathogens [33] and many of the major types of drug resistance that are encountered in the clinic [34] . 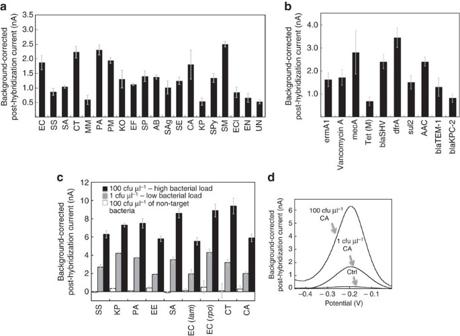Figure 3: Validation of pathogen and antibiotic-resistance probes. (a) Background-corrected post-current values for pathogen probe set. Sensors were challenged with 1 nM of a synthetic DNA complement and the signal generated was compared with that obtained with a 100-nM solution of a non-complementary DNA sequence to obtain the background-corrected value. (b) Background-corrected post-current values for antibiotic-resistance probe set. Sensors were challenged with 1 nM of a synthetic DNA complement, and these signals were compared with those obtained with a 100-nM solution of a non-complementary DNA sequence to obtain the background-corrected value. (c) Pathogen probes validated versus bacterial lysates (EC,E. coli; SS,S. saprophyticus; SA,S. aureus;. CT,C. trachomatis; MM,M. morganii; PA,P. aeruginosa; PM,P. mirabilis; KO,K. oxytoca; EF,E. faecalis; SP,S. pneumonia; AB,A. baumannii; Sag,S. agalactiae; SE,S. epidermis; CA,C. albicans; KP,K. pneumonia; SP,S. pyogenes; Spy,S. pyogenes; SM,S. marescens; ECl,E. cloacae; EN,enterobactergenus; UN, universal bacteria probe). Error bars reflect s.d. collected from data sets obtained with >3 independent chips. (d) Representative differential pulse voltammograms (DPVs) obtained for a control sample (Ctrl), a lysate containing 1 cfu μl−1, and a lysate containing 100 cfu μl−1. Figure 3: Validation of pathogen and antibiotic-resistance probes. ( a ) Background-corrected post-current values for pathogen probe set. Sensors were challenged with 1 nM of a synthetic DNA complement and the signal generated was compared with that obtained with a 100-nM solution of a non-complementary DNA sequence to obtain the background-corrected value. ( b ) Background-corrected post-current values for antibiotic-resistance probe set. Sensors were challenged with 1 nM of a synthetic DNA complement, and these signals were compared with those obtained with a 100-nM solution of a non-complementary DNA sequence to obtain the background-corrected value. ( c ) Pathogen probes validated versus bacterial lysates (EC, E. coli ; SS, S. saprophyticus ; SA, S. aureus ;. CT, C. trachomatis ; MM, M. morganii ; PA, P. aeruginosa ; PM, P. mirabilis ; KO, K. oxytoca ; EF, E. faecalis ; SP, S. pneumonia ; AB, A. baumannii ; Sag, S. agalactiae ; SE, S. epidermis ; CA, C. albicans ; KP, K. pneumonia ; SP, S. pyogenes ; Spy, S. pyogenes ; SM, S. marescens ; ECl, E. cloacae ; EN, enterobacter genus; UN, universal bacteria probe). Error bars reflect s.d. collected from data sets obtained with >3 independent chips. ( d ) Representative differential pulse voltammograms (DPVs) obtained for a control sample (Ctrl), a lysate containing 1 cfu μl −1 , and a lysate containing 100 cfu μl −1 . Full size image We used our multiplexed chips to achieve the parallelized assessment of 30 probes for pathogens and antibiotic-resistance markers ( Fig. 3a ). The pathogen probes were targeted against either the RNA polymerase β mRNA ( rp o β ), or a ribosomal RNA, and the antibiotic-resistance probes were targeted against known sequences correlated with drug deactivation. To screen sequences for specificity, we compared the response obtained from a solution containing a 1-nM concentration of a complementary target with the response from a solution containing a 100-nM concentration of a non-complementary target. The background-subtracted current generated was then analysed, and for the large majority of the probes that were tested the current obtained was greater than baseline by three standard deviations. However, it is noteworthy that the amount of current generated with each probe varies for the different probes. Nonetheless, the magnitude of current generated for each probe was highly reproducible and hence, despite this effect, the approach can be used for specific pathogen detection. The sensitivity of sensors modified with these probes was then tested against a panel of pathogens amenable to culture ( Fig. 3c ). Unpurified bacterial lysates containing 1 cfu μl −1 and 100 cfu μl −1 were incubated with the sensors, and electrochemical signals were compared with those obtained when the same sensor type was exposed to 100 cfu μl −1 of non-target bacteria ( Escherichia coli for each trial, except for those testing the sensitivity of the E. coli probes, where Staphylococcus saprophyticus was used). The signals obtained for each pathogen differed, which likely reflects idiosyncratic nucleic acid structures, but in each case excellent sensitivity and specificity were obtained using samples that have undergone minimal processing. In each case, the signals obtained with solutions containing 1 cfu μl −1 were greater by a factor of at least three standard deviations relative to background signals, indicating that the limits of detection reside at or below this concentration. The detection limit obtained here of 1 cfu μl −1 is clinically significant. Many applications in infectious disease testing—including testing of swab samples for health-care-associated infections or sexually transmitted infections, or the testing of urine for infectious pathogens—yield samples that contain concentrations higher than 1 cfu μl −1 . This detection and speed combination also approaches the diffusional limits for large molecules in static solutions [30] . Multiplexed detection of urinary tract infection pathogens The SCC was then put to the ultimate test: the analysis of samples containing clinically relevant concentrations of pathogens for panels of markers. SCCs were functionalized simultaneously using nine different probes ( Fig. 4a ) and were challenged with bacterial lysates at 100 cfu μl −1 . Chips were first challenged with lysates of E. coli , the most common urinary tract infection-causing pathogen ( Fig. 4b ). The response of sensors modified with the E. coli probe targeted against the RNA polymerase gene ( rpoβ ) was significant, whereas no other probes showed significant response to the lysate. We also challenged chips prepared with the same sensors and probes with a form of antibiotic-resistant E. coli that contains the β-lactamase ( β-lac ) gene ( Fig. 4c ). With this sample, only EC and β-lactamase sensors exhibited a significant response, indicating that the SCC can classify pathogens and detect antibiotic resistance simultaneously. SCCs were also challenged with lysates of Staphylococcus aureus to confirm successful detection of Gram-positive pathogens ( Fig. 4d ). Only electrodes functionalized with SA probe showed a significant electrochemical response. In addition, we challenged chips with a mixture of S. aureus and antibiotic-resistant E. coli (+ β-lac ) to evaluate the performance of chips brought into contact with several analytes producing a positive response (Fig. 4e ). Only electrodes functionalized with matching probes exhibited significant electrochemical responses to the mixed lysed sample. These results illustrate that the multiplexing provided by solution-based circuits enables the parallelized detection of multiple analytes at clinically relevant levels. 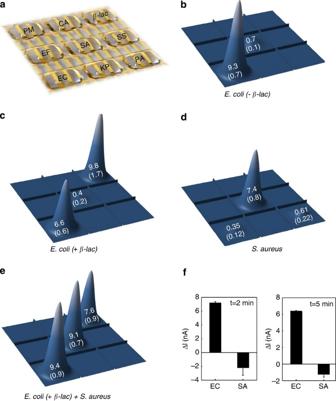Figure 4: Multiplexed pathogen and antibiotic-resistance testing on an SCC. (a) Arrangement of sensors on a 100-plexed SCC. (b) Response of SCC challenged with 100 cfu μl−1E. coli. (−β-lac). (c) Response of SCC challenged with 100 cfu μl−1E. coli. (+β-lac). (d) Response of SCC challenged with 100 cfu μl−1S. aureus. (e) Response of SCC challenged with 100 cfu μl−1S. aureus+E. coli(+β-lac) bacterial lysate. (f) Response of SCC at 2 min and 5 min challenged withE. colilysates at 100 cfu μl−1. Figure 4: Multiplexed pathogen and antibiotic-resistance testing on an SCC. ( a ) Arrangement of sensors on a 100-plexed SCC. ( b ) Response of SCC challenged with 100 cfu μl −1 E. coli. (−β-lac) . ( c ) Response of SCC challenged with 100 cfu μl −1 E. coli . (+ β-lac ). ( d ) Response of SCC challenged with 100 cfu μl −1 S. aureus . ( e ) Response of SCC challenged with 100 cfu μl −1 S. aureus + E. coli (+ β-lac ) bacterial lysate. ( f ) Response of SCC at 2 min and 5 min challenged with E. coli lysates at 100 cfu μl −1 . Full size image As a final test of the utility of the SCC, we investigated whether very short hybridization times could be used to enable very rapid bacterial detection ( Fig. 4f ). We investigated the evolution of signals that could be detected on chip with a 2- and 5-min hybridization, and determined that a pathogen-specific response could be obtained even with the shortest time studied. These results indicate that SCCs can be used for highly multiplexed pathogen detection, and can also be used to deliver the very rapid results needed to make diagnostic information clinically actionable. Using the simple idea that solution-based circuits could be harnessed on chip to enhance the level of multiplexing that could be achieved on a passive chip, we created a new method for electrochemical multiplexing. Compared with complicated and expensive active electronics on the surface of silicon, this approach has significant advantages for the development of low-cost diagnostic tools. A simple six-step fabrication approach, where most of the steps were performed using transparency masks and low-grade glass was used as a substrate, is advantageous over more involved protocols used to create active silicon electronics. The approach reported herein is scalable in that it could be deployed to produce chips with higher levels of multiplexing than shown here. Given the current capabilities of photolithography and technologies that can be used to deliver probe molecules to high-density arrays, thousands of sensors could be addressed using the solution circuit strategy. The development of strategies to maintain the large number of liquid channels would represent the greatest challenge in realizing this level of multiplexing. The sensor technology used here, which relies on the electrodeposition of microscale, three-dimensional sensors, is a powerful tool in the analysis of complex samples. It has been shown to perform well in the presence of blood [23] and urine [25] , and can also discriminate single base changes in sequence [35] . As demonstrated here, it is compatible with unpurified bacterial lysates and, therefore, is easily integrated for sample-to-answer testing. These features provide a significant advantage over gold standard molecular testing methods, such as the PCR, which typically requires sample clean-up and the use of costly enzymatic reagents. It is also compatible with samples ranging from microlitres to millilitres, which broadens the potential clinical utility. Here we have demonstrated that in addition to possessing these features, it can also be used with a highly multiplexed format if the solution circuit approach is used to contact the sensors. The solution-based circuit chip, as it yields rapid and accurate information on the identity and antibiotic resistance of pathogens, represents a significant advance in the field of biomolecular sensing. Multiplexed chip fabrication Multiplexed chips were fabricated in house on plain glass substrates obtained from Telic Company (Valencia, CA). The substrates are precoated with 5 nm Cr followed by 50 nm Au and positive photoresist (AZ1600). The common WEs were imaged using standard contact lithography and etched using Au and Cr wet etchants, followed by removal of the positive photoresist. A negative photoresist SU-8 2002 was spin coated at 5,000 r.p.m. for 30 s and the aperture layer was imaged into the surface. A positive photoresist S1811 was spin coated on the surface and imaged to act as a lift-off layer. The AUX/REF electrodes (5 nm Cr–50 nm Au) were fabricated onto the surface using standard e-beam evaporation followed by lift-off by sonication in acetone. The probe well layer was created using SU-8 2002 spin coated at 3,000 r.p.m. for 30 s. A thicker liquid channel layer was fabricated with SU-8 3025 at 2,000 r.p.m. for 30 s. A plasma etch mask layer with openings defined for the probe wells was patterned on the surface using SPR 7.0 at 2,000 r.p.m. for 30 s. Chips were diced in house using a standard straight edge scriber. Before electroplating, chips were O 2 plasma etched in a Samco-RIE-1C reactive ion etcher at 15 W for 15 s to create a hydrophilic probe well area. The core structure of the nanostructured microelectrodes was fabricated by electroplating chips in a solution of 50 mM HAuCl 4 and 0.5 M HCl at 0 mV for 100 s. The nanostructured surface of the nanostructured microelectrodes was generated by electrodeposition of a Pd coating in a solution of 5 mM PdCl 2 and 0.5 HClO 4 at −250 mV for 10 s. Electrochemical chip characterization Ferricyanide was used to evaluate the electrochemical characteristics of the multiplexed chip. Standard cyclic voltammetry in 2 mM Fe(CN) 6 3− in 0.1 × PBS scanned from 50 mV to −300 mV at 100 mV s −1 versus on-chip Au AUX/REF was performed on the surface of chips of similar layout that have WEs that are individually addressed versus the multiplexed chips with solution circuits. In addition, ferricyanide crosstalk was evaluated by filling a single channel with 2 mM Fe(CN) 6 3− in 0.1 × PBS and adjacent channels with 0.1 × PBS. Differential pulse voltammetry from 50 mV to −300 mV was performed in the ferricyanide-containing channel and adjacent channels without ferricyanide. Spectroscopic chip characterization The MB crosstalk experiment was performed on the surface of SCCs by first loading each liquid channel with a solution of 100 μM MB and 50 mM NaCl. Chips were placed in a humidity chamber where the middle lane WEs and AUX/REF was held under bias for 1 h at −650 mV, which is a sufficient potential for reduction of MB. The MB in each channel was then diluted by a factor of 10 and the corresponding absorbance was measured with a ultraviolet–visible spectrophotometer. Electrochemical assay crosstalk evaluation Probe wells on the surface of multiplexed chips were used to functionalize with target-specific PNA probes. Each well was filled with 1.5 μl of complementary or non-complementary probe solution initially heated to 60 °C for 5 min, containing 100 nM probe and 900 nM mercaptohexanol, and was incubated directly on chip for 30 min at room temperature. Chips were washed with 0.1 × PBS twice for 5 min after probe deposition, and an initial DPV background scan in electrocatalytic solution (10 μM Ru(NH 3 ) 6 3+ and 4 mM Fe(CN) 6 3− in a 0.1 × PBS) was performed. Chips were then hybridized with 10 nM complementary target in 1 × PBS for 30 min at 37 °C. Chips were washed with 0.1 × PBS twice for 5 min after target hybridization and differential pulse voltammetry hybridization scan in electrocatalytic solution was performed. Identification of pathogen-specific probes A list of potential probes based on the rpoβ gene sequences of the bacteria under study was first generated. All sequences were obtained from the NCBI Nucleotide Database. For a given bacterial sequence, a BLAST search was performed to identify the rpoβ sequence of the most similar bacterial species that could potentially cross-hybridize. This sequence was retrieved and aligned with the targeted bacterial sequence using CLUSTALW2. A computer script was used to identify regions of greatest variability, as they can be used to best differentiate the target species from non-target species. Potential rpoβ probes that could cross-hybridize with non-target molecules in patient samples were eliminated first. Other probe characteristics, such as secondary structure melting temperature, were also analysed to ensure optimal specificity. If suitable probes could not be identified targeting the rpoβ mRNA, then the 16S rRNA ( Morganella morganii , Pseudomonas aeruginosa , Enterobacteria family and universal probe) or the 28S rRNA ( Candida albicans ) was used as a target instead. Synthesis of probes Synthesis of PNA probes was performed in house using a Protein Technologies Prelude peptide synthesizer. The following pathogen probe sequences (NH 2 -Cys-Gly-Asp SEQUENCE Asp- CONH 2 ) that are specific to mRNA targets were synthesized: E. coli , 5′-ATC-TGC-TCT-GTG-GTG-TAG-TT-3′; Proteus mirabilis , 5′-AAG-CGA-GCT-AAC-ACA-TCT-AA-3′; S. saprophyticus , 5′-AAG-TAA-GAC-ATT-GAT-GCA-AT-3′; S. aureus , 5′-CCA-CAC-ATC-TTA-TCA-CCA-AC-3′; Klebsiella pneumoniae , 5′-GTT-TAG-CCA-CGG-CAG-TAA-CA-3′; M. morganii , 5′-CGC-TTT-GGT-CCG-AAG-ACA-TTA-T-3′; P. aeruginosa , 5′-CCC-GGG-GAT-TTC-ACA-TCC-AAC-TT-3′; K. oxytoca , 5′-CCA-GTA-GAT-TCG-TCA-ACA-TA-3′; Serratia marescens , 5′-TGC-GAG-TAA-CGT-CAA-TTG-ATG-A-3′; Enterococcus faecalis , 5′-CGA-CAC-CCG-AAA-GCG-CCT-TT-3′; Acinetobacter baumannii , 5′-CGT-CAA-GTC-AGC-ACG-TAA-TG-3′; Streptococcus pyogenes , 5′-TCT-TGA-CGA-CGG-ATT-TCC-AC-3′; Streptococcus agalactiae , 5′-GTT-CAG-TAA-CTA-CAG-CAT-AA-3′; Staphylococcus epidermidis , 5′-AAA-TAA-CTC-ATT-GAG-GCA-AC-3′; Enterobacter cloacae , 5′-TCA-ACG-TAA-TCT-TTC-GCG-GC-3′; Streptococcus pneumoniae , 5′-GTT-ACG-ACG-CGA-TCT-GGA-TC-3′; Providencia stuartii , 5′-GCC-AAG-TGC-CAA-TTC-ACC-TAG-3′; C. albicans , 5′-GCT-ATA-ACA-CAC-AGC-AGA-AG-3′; Chlamydia trachomatis , 5′-TGC-ATT-TGC-CGT-CAA-CTG-3′; Enterobacteriaceae, 5′-ACT-TTA-TGA-GGT-CCG-CTT-GCT-CT-3′; and Universal bacteria probe, 5′-GGT-TAC-CTT-GTT-ACG-ACT-T-3′. After synthesis, all probes were stringently purified using reverse-phase HPLC. Excitation coefficients were calculated from http://www.panagene.com and concentrations of probe molecules were determined by measuring absorbance at 260 nm with a NanoDrop spectrophotometer. Preparation of bacterial samples and lysis The following bacterial strains were used in this study: K. pneumoniae ATCC 27799, E. coli K12 ATCC 33876, E. col i Invitrogen 18265-017, S. saprophyticus ATCC 15305, P. aeruginosa PAO1, E. faecalis ATCC 29212, S. aureus , C. trachomatis and C. albicans. All bacteria were grown in the appropriate growth media and conditions. Approximate quantification of bacteria was performed by measuring the optical density at 600 nm with an Agilent 8453 ultraviolet–visible spectrometer. After the desired population was reached, the growth media was replaced with 1 × PBS. Lysis of bacteria was performed utilizing the Claremont BioSolutions OmniLyse rapid cell lysis kit. Probe validation Probe solutions were initially heated to 60 °C for 5 min before deposition, and contained 100 nM probe and 900 nM mercaptohexanol. Deposition was carried out for 30 min at room temperature. Chips were washed with 0.1 × PBS twice for 5 min after probe deposition and chips were then challenged with a non-complementary oligomer at 100 nM in 1 × PBS for 30 min. Chips were washed with 0.1 × PBS twice for 5 min, and then an initial non-complementary DPV background scan was performed in electrocatalytic solution (10 Ru(NH 3 ) 6 3+ and 4 mM Fe(CN) 6 3− in a 0.1 × PBS). Chips were then hybridized with 1 nM complementary target in 1 × PBS for 30 min at 37 °C. Chips were washed with 0.1 × PBS twice for 5 min after target hybridization and a DPV in electrocatalytic solution was then performed. A similar protocol was followed for lysate testing. Chips were hybridized with lysates in 1 × PBS for 30 min at 37 °C. Chips were washed with 0.1 × PBS twice for 5 min after target hybridization and DPV hybridization scan in electrocatalytic solution was performed. Multiplexed bacterial lysate experiments Multiplexed chips for bacterial lysate testing were functionalized with nine probes using nine probe wells. Probe solutions were initially heated to 60 °C for 5 min, and contained 100 nM probe and 900 nM mercaptohexanol that was incubated directly on chip for 30 min at room temperature. Chips were washed with 0.1 × PBS twice for 5 min after probe deposition and an initial DPV background scan was collected in electrocatalytic solution. Multiplexed chips were then hybridized with individual and mixed lysates at 100 cells per μl in 1 × PBS for 30 min at 37 °C in a 200-μl volume. How to cite this article: Lam, B. et al. Solution-based circuits enable rapid and multiplexed pathogen detection. Nat. Commun. 4:2001 doi: 10.1038/ncomms3001 (2013).